A short acidic motif in ARF guards against mitochondrial dysfunction and melanoma susceptibility ARF is a small, highly basic protein that can be induced by oncogenic stimuli and exerts growth-inhibitory and tumour-suppressive activities through the activation of p53. Here we show that, in human melanocytes, ARF is cytoplasmic, constitutively expressed, and required for maintaining low steady-state levels of superoxide under conditions of mitochondrial dysfunction. This mitochondrial activity of ARF is independent of its known autophagic and p53-dependent functions, and involves the evolutionarily conserved acidic motif GHDDGQ, which exhibits weak homology to BCL-2 homology 3 (BH3) domains and mediates interaction with BCL-xL—an important regulator of mitochondrial redox homeostasis. Melanoma-predisposing CDKN2A germline mutations, which affect conserved glycine and aspartate residues within the GHDDGQ motif, impair the ability of ARF to control superoxide production and suppress growth of melanoma cells in vivo . These results reveal an important cell-protective function of ARF that links mitochondrial dysfunction and susceptibility to melanoma. The ARF tumour suppressor (p14 ARF in humans, p19 Arf in mice) is silenced or genetically lost in a broad spectrum of human cancers. It is widely accepted that ARF is a predominantly nucleolar protein that can be induced in response to oncogenic insults [1] . Under normal physiological conditions, the expression of ARF protein has been detected only in the developing eye and in mitotically dividing spermatogonia [2] , [3] . ARF is a highly basic protein that has no obvious structural elements, but contains subcellular localization signals and conserved motifs required for interaction with other proteins [1] . The best understood function of ARF is the ability to inhibit growth of malignant or oncogenically stressed cells by regulating the p53 pathway through binding to MDM2 (ref. 4 ). In addition, ARF exerts p53-independent tumour-suppressive activities [1] , [5] . The spectrum of cancers developing in mice lacking Arf , Trp53 and Mdm2 is wider than in mice lacking Trp53 and Mdm2 (ref. 5 ), and reconstitution of ARF can arrest proliferation of Trp53 -null cells [6] , [7] . Numerous reports based on cell culture experiments have implicated ARF in the regulation of diverse cellular processes, including ribosomal biosynthesis, the DNA damage response pathway, cell cycle arrest, senescence, apoptosis and autophagy [8] , [9] , [10] , [11] , [12] , suggesting that the tumour-suppressive functions of ARF may be both cell type and context dependent. ARF is encoded by the CDKN2A locus, which also encodes p16 (INK4A), a potent tumour suppressor that acts through the retinoblastoma pathway. CDKN2A has been identified as the major high-penetrance cutaneous melanoma predisposition locus, accounting for 40% of multiple-case melanoma families [13] , [14] , [15] . The vast majority of CDKN2A germline mutations are predicted to affect p16, with less than half of these mutations also affecting ARF [14] . Nevertheless, several lines of evidence point to an independent role of ARF as a suppressor of melanoma, including the segregation of ARF-selective mutations in melanoma-prone families [14] , [15] , [16] , [17] , [18] , [19] , and the fact that mutations affecting both p16 and ARF confer a higher penetrance than mutations affecting p16 alone [20] , [21] . Activating mutation of BRAF is a common initiating event in melanoma development that leads to constitutive activation of the RAS–RAF–MEK–ERK signal transduction pathway. Despite the induction of ARF expression by a variety of oncogenic stimuli, including MYC [22] , previous studies have failed to identify a role of ARF in inducing senescence as a first-line defence against oncogenic BRAF in melanocytes [23] , [24] . Why ARF mutations predispose to melanoma remains unclear. Here we have identified an ARF-mediated mechanism required to maintain low steady-state levels of superoxide in cells containing injured or dysfunctional mitochondria. The amino acid residues found to be responsible for this function of ARF are selectively targeted in familial melanoma. ARF translocates to dysfunctional mitochondria To identify a normal physiological function of ARF of potential relevance to melanoma susceptibility, we chose replicative senescence of human melanocytes as a model for our initial investigations. Examination of ARF expression in these cells using carefully validated antibodies ( Supplementary Fig. 1 ) and reverse transcriptase-PCR led to a number of unexpected findings. First, ARF was constitutively expressed throughout the entire cellular lifespan and showed an increased expression after ~25 population doublings (PD; Fig. 1a and Supplementary Fig. 2 ). Second, ARF was consistently detected in the cytoplasmic compartment and, unlike p16, not detectable in the nucleus at any stage ( Fig. 1a ). As a control, the same ARF antibody detected nuclear ARF in non-melanocytic cells ( Supplementary Fig. 1 ). The subcellular localization of ARF has been proposed to be regulated by nucleophosmin (NPM/B23) (refs 25 , 26 ), a known interaction partner for ARF [27] . Consistent with this notion, we found a correlation between the expression levels of NPM and the localization of ARF in melanocytic cells. Specifically, immunoblot analysis showed that NPM is expressed at low levels in normal melanocytes, whereas it is expressed at high levels in ARF-expressing melanoma cell lines where ARF shows both nuclear and cytoplasmic localization ( Supplementary Fig. 3a ). Furthermore, the increased expression of cytoplasmic ARF during replicative aging of melanocytes correlated with a decrease in NPM expression ( Supplementary Fig. 3b ). Finally, depletion of NPM in ARF-expressing melanoma cells induced a shift from nuclear to cytoplasmic localization of ARF ( Supplementary Fig. 3c ). These data suggest that the restriction of ARF to the cytoplasmic compartment in melanocytes can be attributed to the low levels of NPM in these cells. 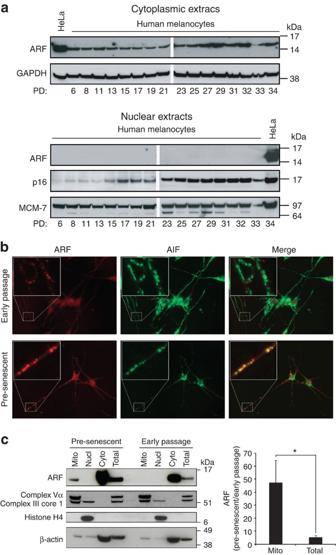Figure 1: Cytoplasmic and mitochondrial localization of endogenous ARF in human melanocytes undergoing replicative senescence. (a) Representative immunoblot analysis of nuclear (45 μg) and cytoplasmic (100 μg) extracts. (b) Immunofluorescence staining of early-passage (<15 PD) and pre-senescent (30–33 PD) melanocytes using antibodies against ARF (red) and the mitochondrial protein, apoptosis-inducing factor (AIF; green). (c) Left, immunoblot analysis of ARF in total cell lysates (Total) and in cytoplasmic (Cyto), mitochondrial (Mito) and nuclear (Nucl) fractions from early-passage and pre-senescent melanocytes. Right, relative ARF levels in mitochondrial fractions and total cell lysates. Data are based on three independent experiments and corrected for differences in the levels of complex V α-subunit (control for loading) and β-actin. Error bars indicate s.d.,n=3. ThePvalue was obtained using a pairedt-test; *P<0.05. Figure 1: Cytoplasmic and mitochondrial localization of endogenous ARF in human melanocytes undergoing replicative senescence. ( a ) Representative immunoblot analysis of nuclear (45 μg) and cytoplasmic (100 μg) extracts. ( b ) Immunofluorescence staining of early-passage (<15 PD) and pre-senescent (30–33 PD) melanocytes using antibodies against ARF (red) and the mitochondrial protein, apoptosis-inducing factor (AIF; green). ( c ) Left, immunoblot analysis of ARF in total cell lysates (Total) and in cytoplasmic (Cyto), mitochondrial (Mito) and nuclear (Nucl) fractions from early-passage and pre-senescent melanocytes. Right, relative ARF levels in mitochondrial fractions and total cell lysates. Data are based on three independent experiments and corrected for differences in the levels of complex V α-subunit (control for loading) and β-actin. Error bars indicate s.d., n =3. The P value was obtained using a paired t -test; * P <0.05. Full size image While ARF showed a uniform distribution throughout the cytoplasm of early-passage melanocytes (<15 PD), it co-localized with mitochondria in pre-senescent cells (30–33 PD; Fig. 1b and Supplementary Fig. 4 ). This age-dependent mitochondrial enrichment of ARF was greater than the corresponding increase in total ARF ( Fig. 1c ). As cellular senescence and aging are associated with deterioration of mitochondrial function [28] , [29] , [30] , we asked if mitochondrial dysfunction could provide the signal that triggered translocation of ARF to mitochondria during replicative senescence. Consistent with this idea, pre-senescent and senescent cells contained dysfunctional mitochondria according to several criteria, including reduced signals from MitoTracker Red and DiOC 6 (fluorescent dyes that accumulate in mitochondria with an intact membrane potential (ΔΨ m )), reduced ATP production, activation of AMP-activated protein kinase (AMPK; a sensor of bioenergetic stress), lower mitochondrial DNA (mtDNA) copy number and a tendency towards lower levels of the mitochondrial protein cyclophilin D ( Fig. 2a,b and Supplementary Figs 5 and 6 ). Furthermore, pre-senescent cells had a lower coupling efficiency and lower respiratory control ratio (RCR) values than early-passage cells, as measured by the oxygen consumption rate (OCR) ( Fig. 2c–e ). A lower RCR has also been observed in senescent fibroblasts [31] . 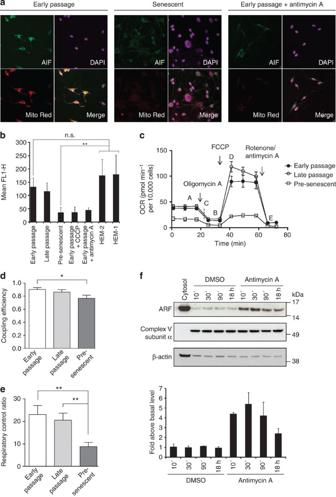Figure 2: Metabolic differences associated with replicative senescence of human epidermal melanocytes. (a) MitoTracker Red staining in early-passage (<15 PD) and senescent melanocytes and in early-passage melanocytes treated overnight with antimycin A (25 μM). Cells were co-stained for AIF (green) and 4′,6-diamidino-2-phenylindole (DAPI; violet). (b) ΔΨmmeasured by DiOC6(3) staining and flow cytometric analysis in late-passage (>15 PD) and pre-senescent (30–33 PD) melanocytes, early-passage melanocytes treated with the mitochondrial uncoupler CCCP (20 μM, 20 min) or antimycin A (25 μM, overnight) and ARF/p16-depleted melanocytes (HEM-1 and HEM-2). Error bars indicate s.d.,n=3. (c) OCR in early-passage, late-passage and pre-senescent melanocytes following sequential addition of oligomycin (1 μM), carbonylcyanide-p-trifluoromethoxyphenylhydrazone (FCCP, 2.5 μM) and a mixture of antimycin A (2.5 μM) and rotenone (2.5 μM). Different states of mitochondrial respiration are indicated; basal respiration (A), proton leak (B), oligomycin-sensitive respiration (C=A−B), maximal respiratory rate (D) and non-mitochondrial respiration (E). (d) Calculation of the coupling efficiency of oxidative phosphorylation (C/A) and (e) the RCR (D/B) in early-passage, late-passage and pre-senescent melanocytes. Error bars (c–e) indicate s.d. (n=6) from one experiment, representative of two independent experiments. (f) Top, immunoblot analysis of ARF in mitochondrial extracts from early-passage melanocytes following treatment with antimycin A (5 μM). Bottom, relative levels of ARF in mitochondrial fractions after antimycin A treatment. Data are based on three independent experiments and corrected for differences in the levels of complex V α-subunit and β-Actin. Error bars indicate s.d.,n=3.Pvalues (b,d,e) were determined with one-way ANOVA, using Tukey’s multiple comparisons test (*P<0.05; **P<0.01). Figure 2: Metabolic differences associated with replicative senescence of human epidermal melanocytes. ( a ) MitoTracker Red staining in early-passage (<15 PD) and senescent melanocytes and in early-passage melanocytes treated overnight with antimycin A (25 μM). Cells were co-stained for AIF (green) and 4′,6-diamidino-2-phenylindole (DAPI; violet). ( b ) ΔΨ m measured by DiOC 6 (3) staining and flow cytometric analysis in late-passage (>15 PD) and pre-senescent (30–33 PD) melanocytes, early-passage melanocytes treated with the mitochondrial uncoupler CCCP (20 μM, 20 min) or antimycin A (25 μM, overnight) and ARF/p16-depleted melanocytes (HEM-1 and HEM-2). Error bars indicate s.d., n =3. ( c ) OCR in early-passage, late-passage and pre-senescent melanocytes following sequential addition of oligomycin (1 μM), carbonylcyanide-p-trifluoromethoxyphenylhydrazone (FCCP, 2.5 μM) and a mixture of antimycin A (2.5 μM) and rotenone (2.5 μM). Different states of mitochondrial respiration are indicated; basal respiration (A), proton leak (B), oligomycin-sensitive respiration (C=A−B), maximal respiratory rate (D) and non-mitochondrial respiration (E). ( d ) Calculation of the coupling efficiency of oxidative phosphorylation (C/A) and ( e ) the RCR (D/B) in early-passage, late-passage and pre-senescent melanocytes. Error bars ( c – e ) indicate s.d. ( n =6) from one experiment, representative of two independent experiments. ( f ) Top, immunoblot analysis of ARF in mitochondrial extracts from early-passage melanocytes following treatment with antimycin A (5 μM). Bottom, relative levels of ARF in mitochondrial fractions after antimycin A treatment. Data are based on three independent experiments and corrected for differences in the levels of complex V α-subunit and β-Actin. Error bars indicate s.d., n =3. P values ( b , d , e ) were determined with one-way ANOVA, using Tukey’s multiple comparisons test (* P <0.05; ** P <0.01). Full size image To test whether ARF responds to an acute state of mitochondrial dysfunction, we treated early-passage melanocytes with antimycin A (a mitochondrial complex III inhibitor), oligomycin A (an ATP synthase inhibitor), CCCP (a chemical uncoupler) or a combination of oligomycin A and CCCP. As shown in Fig. 2f and Supplementary Fig. 7 , treatment with antimycin A or a combination of oligomycin A and CCCP caused immediate accumulation of ARF in the mitochondrial fraction. Previous studies have shown that inhibition of oncogenic BRAF E600 in melanoma cells causes a redirection of metabolism towards the compensatory use of oxidative phosphorylation [32] , [33] . To study if a metabolic shift could lead to the activation of ARF by unmasking mitochondrial dysfunction inherently present in melanoma cells, we treated ARF-proficient melanoma cells with the glycolysis inhibitor 2-deoxy- D -glucose (2-DG). As expected, this treatment induced a metabolic shift and a reduction in ATP levels ( Fig. 3a,b ). Importantly, ARF accumulated in the mitochondrial fraction of these cells 18–24 h after induction, as determined by biochemical fractionation ( Fig. 3c ) and super-resolution-structured illumination microscopy (SR-SIM; Supplementary Fig. 8 ). Thus, mitochondrial dysfunction, whether age-related, chemically induced or inherently present in cancer cells, could trigger mitochondrial translocation of ARF. 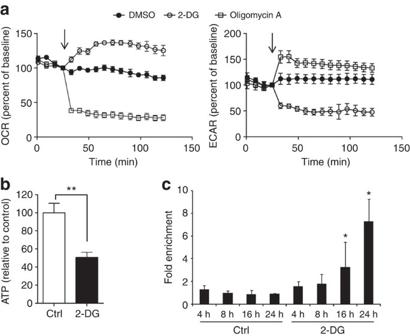Figure 3: Translocation of ARF to mitochondria in melanoma cells undergoing a metabolic shift. (a) OCR and ECAR in FM55-M2 cells following addition of 2-DG (10 mM), oligomycin A (1 μM) or dimethylsulphoxide (DMSO). Error bars indicate s.d. (n=8) from one experiment, representative of three independent experiments. (b) ATP levels in FM55-M2 cells treated for 4 h with 2-DG and shown relative to DMSO-treated cells (control). Error bars indicate s.d.,n=5.Pvalue was determined by Student’st-test. (c) Time-dependent enrichment of ARF in digitonin-insoluble/triton-soluble organelle fractions of FM55-M2 cells treated with 2-DG. Data are based on three independent experiments and corrected for differences in the levels of mitochondrial protein and LAMIN B (a marker of contamination with nuclear proteins). Error bars indicate s.d.,n=3.Pvalues were determined with one-way ANOVA, using Tukey’s multiple comparisons test. *P<0.05; **P<0.01. Figure 3: Translocation of ARF to mitochondria in melanoma cells undergoing a metabolic shift. ( a ) OCR and ECAR in FM55-M2 cells following addition of 2-DG (10 mM), oligomycin A (1 μM) or dimethylsulphoxide (DMSO). Error bars indicate s.d. ( n =8) from one experiment, representative of three independent experiments. ( b ) ATP levels in FM55-M2 cells treated for 4 h with 2-DG and shown relative to DMSO-treated cells (control). Error bars indicate s.d., n =5. P value was determined by Student’s t -test. ( c ) Time-dependent enrichment of ARF in digitonin-insoluble/triton-soluble organelle fractions of FM55-M2 cells treated with 2-DG. Data are based on three independent experiments and corrected for differences in the levels of mitochondrial protein and LAMIN B (a marker of contamination with nuclear proteins). Error bars indicate s.d., n =3. P values were determined with one-way ANOVA, using Tukey’s multiple comparisons test. * P <0.05; ** P <0.01. Full size image ARF reduces mitochondrial respiratory capacity The association of endogenous ARF with dysfunctional mitochondria in melanocytes undergoing replicative senescence prompted a series of stable knockdown experiments to investigate whether senescence and low mitochondrial activity were causes or consequences of ARF translocation. In accordance with previous studies demonstrating a key role of p16 in melanocyte senescence [34] , we were unable to propagate long-term cultures of ARF-depleted melanocytes without concomitant depletion of p16. In contrast, cultures stably depleted of both proteins had an extended lifespan ( Supplementary Fig. 9 ), and finally arrested with high levels of apoptosis, indicative of cellular crisis, but with no signs of senescence ( Supplementary Fig. 10 ). Selective depletion of p16 also resulted in senescent cultures (data not shown), suggesting that ARF constitutes an important component of the replicative senescence barrier in melanocytes. Late-passage ARF/p16-depleted cells showed marked differences in mitochondrial activity compared with their normal pre-senescent and senescent counterparts, including the ability to maintain a ΔΨ m similar to or even higher than that present in early-passage cells ( Fig. 2b ). Hence, the loss of mitochondrial activity observed in normal pre-senescent melanocytes appeared to be mediated by ARF. This was further corroborated by experiments performed in pre-senescent cultures, where even a modest reduction in ARF levels resulted in improved maximal respiratory rate and a higher RCR, as measured by a higher oxygen consumption following treatment with the chemical uncoupler FCCP ( Fig. 4a–d ). These data showed that ARF causes reduced respiratory capacity in normal pre-senescent melanocytes, in accordance with the observed changes in ΔΨ m . The levels of p16 remained stable in pre-senescent cells depleted of ARF, suggesting that p16 did not contribute to the observed changes in mitochondrial activity ( Fig. 4a ). 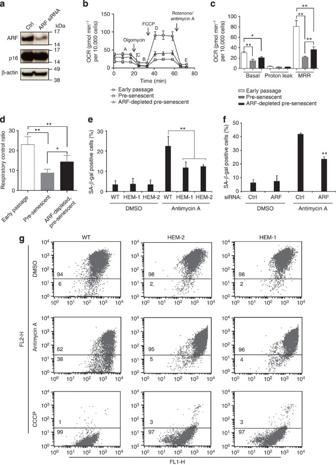Figure 4: Effects of ARF on mitochondrial respiratory capacity, ΔΨmand senescence. (a) Knockdown of ARF in pre-senescent melanocytes (30–33 PD) using short interfering RNA (siRNA) specific to exon 1β. (b) OCR and (c) basic respiratory parameters in early-passage and pre-senescent melanocytes 48 h post transfection with NON-target siRNA or ARF-specific siRNA. OCR was recorded following sequential addition of oligomycin (1 μM), carbonylcyanide-p-trifluoromethoxyphenylhydrazone (FCCP, 2.5 μM) and a mixture of antimycin A (2.5 μM) and rotenone (2.5 μM). Inb, different states of mitochondrial respiration are indicated; basal respiration (A), proton leak (B), oligomycin-sensitive respiration (C=A−B), maximal respiratory rate (D) and non-mitochondrial respiration (E). (d) RCR in early-passage and pre-senescent melanocytes. Error bars (b–d) indicate s.d. (n=6) from one experiment, representative of two independent experiments. (e,f) SA-β-Gal staining after 1 week of treatment with antimycin A (5 μM) or vehicle (DMSO) in normal early-passage (WT) and ARF/p16-depleted (HEM-1 and HEM-2) melanocytes (e), and in early-passage melanocytes transfected twice with non-targeting or ARF-specific siRNAs before drug treatment (f). Error bars indicate s.d.,n=3. (g) ΔΨmmeasured by JC-1 staining and flow cytometric analysis. Shown is the effect of DMSO (90 min), antimycin A (5 μM for 90 min) and CCCP (50 μM, 20 min) in normal early-passage melanocytes and in HEM-1 and HEM-2. Results are representative of two experiments. Numbers refer to percentages of analysed cells above and below the indicated line.Pvalues were determined with one-way ANOVA, using Tukey’s multiple comparisons test. *P<0.05; **P<0.01. Figure 4: Effects of ARF on mitochondrial respiratory capacity, ΔΨ m and senescence. ( a ) Knockdown of ARF in pre-senescent melanocytes (30–33 PD) using short interfering RNA (siRNA) specific to exon 1β. ( b ) OCR and ( c ) basic respiratory parameters in early-passage and pre-senescent melanocytes 48 h post transfection with NON-target siRNA or ARF-specific siRNA. OCR was recorded following sequential addition of oligomycin (1 μM), carbonylcyanide-p-trifluoromethoxyphenylhydrazone (FCCP, 2.5 μM) and a mixture of antimycin A (2.5 μM) and rotenone (2.5 μM). In b , different states of mitochondrial respiration are indicated; basal respiration (A), proton leak (B), oligomycin-sensitive respiration (C=A−B), maximal respiratory rate (D) and non-mitochondrial respiration (E). ( d ) RCR in early-passage and pre-senescent melanocytes. Error bars ( b – d ) indicate s.d. ( n =6) from one experiment, representative of two independent experiments. ( e , f ) SA- β -Gal staining after 1 week of treatment with antimycin A (5 μM) or vehicle (DMSO) in normal early-passage (WT) and ARF/p16-depleted (HEM-1 and HEM-2) melanocytes ( e ), and in early-passage melanocytes transfected twice with non-targeting or ARF-specific siRNAs before drug treatment ( f ). Error bars indicate s.d., n =3. ( g ) ΔΨ m measured by JC-1 staining and flow cytometric analysis. Shown is the effect of DMSO (90 min), antimycin A (5 μM for 90 min) and CCCP (50 μM, 20 min) in normal early-passage melanocytes and in HEM-1 and HEM-2. Results are representative of two experiments. Numbers refer to percentages of analysed cells above and below the indicated line. P values were determined with one-way ANOVA, using Tukey’s multiple comparisons test. * P <0.05; ** P <0.01. Full size image Collectively, the above results indicated that ARF responds to mitochondrial dysfunction by dissipating ΔΨ m and inducing a senescence response. As an independent means for testing this idea, we induced complex III deficiency, which has been shown to induce premature senescence in fibroblasts [35] . Treatment of normal early-passage melanocytes with antimycin A for 1 week induced premature senescence, which was significantly less pronounced in ARF/p16-depleted cultures ( Fig. 4e ) and melanocytes transiently depleted of ARF ( Fig. 4f ). Moreover, antimycin A caused rapid dissipation of ΔΨ m in normal, but not ARF/p16-depleted melanocytes, indicating that the loss of ΔΨ m in response to antimycin A can be attributed to the function of ARF. In contrast, loss of ΔΨ m in response to the mitochondrial uncoupler CCCP was independent of ARF status ( Fig. 4g ). It has been previously shown that the activation of AMPK due to bioenergetic stress accelerates p53-dependent cellular senescence [36] . Consistent with these findings, senescence induced by antimycin A could be rescued by knockdown of p53 ( Supplementary Fig. 11a ). Furthermore, the treatment of melanocytes with antimycin A led to the rapid activation of AMPK and phosphorylation of p53 at serine 15. However, the activation of AMPK and p53 declined in ARF-depleted cells, whereas it persisted in ARF-expressing cells ( Supplementary Fig. 11b ). This observation confirmed that, by dissipating ΔΨ m , ARF potentiates the bioenergetic stress induced by inhibition of oxidative phosphorylation. ARF controls superoxide production A hallmark of mitochondrial dysfunction is increased production of the oxygen radical superoxide anion, a normal by-product of oxidative phosphorylation that is formed at increased rates when the electron transport chain is defective. Once formed, superoxide is converted to other reactive oxygen species (ROS), which can damage cellular components, including mitochondrial and nuclear DNA, activate cellular checkpoints and lead to cell death [30] . Consistent with progressive accumulation of oxidative damage and the ensuing DNA damage signalling in melanocytes, the levels of 8-oxoguanine, γ-H2AX and phosphorylated ATM increased with age ( Supplementary Fig. 12 ). The overall levels of ROS remained relatively stable over the lifespan of these cells ( Fig. 5a ), which could account for the observed accumulation of oxidative damage. Unexpectedly, however, superoxide levels were 10 times lower in senescent than in early-passage melanocytes ( Fig. 5a ). In contrast, ARF/p16-depleted melanocytes had at least twofold higher basal levels of superoxide than normal melanocytes having undergone the same number of PDs ( Fig. 5a ), and the antimycin A-induced increase in superoxide was twofold higher in ARF/p16-depleted melanocytes than in normal cells ( Supplementary Fig. 13 ). Previous studies have implicated p16 in the control of the general levels of cellular ROS [37] . However, the observed increase in superoxide in ARF/p16-depleted cells could be attributed to ARF deficiency alone, as it could be rescued by re-expression of ARF, but not p16 ( Supplementary Fig. 13 ). As expected, ectopic ARF was associated with mitochondria in these cells ( Supplementary Fig. 13 ). Furthermore, increased levels of superoxide could also be rescued by overexpression of ARF in normal melanocytes treated with antimycin A ( Fig. 5b,c ). 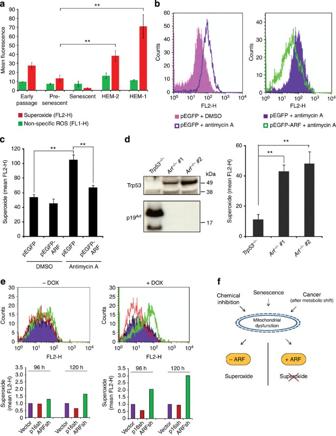Figure 5: ARF-dependent downregulation of superoxide from dysfunctional mitochondria. (a) Detection of non-specific ROS by carboxy-H2DCFDA (green) and superoxide by MitoSOX Red (red) in normal (early-passage, pre-senescent and senescent) and ARF/p16-depleted (HEM-1 and HEM-2) melanocytes. Shown is the mean FL1-H (non-specific ROS) and mean FL2-H (superoxide). (b,c) Fluorescence-activated cell sorting (FACS) analysis showing the downregulation of superoxide following ectopic expression of ARF in early-passage melanocytes. Cells were transfected with pEGFP or pEGFP-ARF vectors and treated with DMSO or antimycin A (5 μM, 90 min). Representative FACS histograms (b) and quantification of mean MitoSOX Red fluorescence from three experiments (c). Data were analysed using one-way ANOVA with Tukeypost hoctests; selected comparisons are shown; **P<0.01. (d) Levels of superoxide in MEFs fromTrp53−/−andArf−/−mice. Left, immublot analysis of Trp53 and p19Arfexpression. Right, mean MitoSOX Red fluorescence from three experiments. (e) FACS analysis of superoxide levels in inducible FM55-M2: TRExE600BRAFsh cells with stable knockdown of p16 (p16sh) or ARF (ARFsh) or mock-transfected (vector). Cells were examined in the absence or presence of doxycycline (DOX) that induces knockdown of BRAFE600and causes a metabolic shift. Top, representative FACS histograms. Bottom, mean MitoSOX Red fluorescence following doxycycline treatment for 96 or 120 h. Data are representative of two independent experiments. (f) Model depicting how ARF controls superoxide production under various conditions of mitochondrial dysfunction. In all graphs, error bars indicate s.d.,n=3.Pvalues were determined with one-way ANOVA, using Tukey’s multiple comparisons test (a,c) or Student’st-test (d). **P<0.01. Figure 5: ARF-dependent downregulation of superoxide from dysfunctional mitochondria. ( a ) Detection of non-specific ROS by carboxy-H 2 DCFDA (green) and superoxide by MitoSOX Red (red) in normal (early-passage, pre-senescent and senescent) and ARF/p16-depleted (HEM-1 and HEM-2) melanocytes. Shown is the mean FL1-H (non-specific ROS) and mean FL2-H (superoxide). ( b , c ) Fluorescence-activated cell sorting (FACS) analysis showing the downregulation of superoxide following ectopic expression of ARF in early-passage melanocytes. Cells were transfected with pEGFP or pEGFP-ARF vectors and treated with DMSO or antimycin A (5 μM, 90 min). Representative FACS histograms ( b ) and quantification of mean MitoSOX Red fluorescence from three experiments ( c ). Data were analysed using one-way ANOVA with Tukey post hoc tests; selected comparisons are shown; ** P <0.01. ( d ) Levels of superoxide in MEFs from Trp53 −/− and Arf −/− mice. Left, immublot analysis of Trp53 and p19 Arf expression. Right, mean MitoSOX Red fluorescence from three experiments. ( e ) FACS analysis of superoxide levels in inducible FM55-M2: TREx E600 BRAFsh cells with stable knockdown of p16 (p16sh) or ARF (ARFsh) or mock-transfected (vector). Cells were examined in the absence or presence of doxycycline (DOX) that induces knockdown of BRAF E600 and causes a metabolic shift. Top, representative FACS histograms. Bottom, mean MitoSOX Red fluorescence following doxycycline treatment for 96 or 120 h. Data are representative of two independent experiments. ( f ) Model depicting how ARF controls superoxide production under various conditions of mitochondrial dysfunction. In all graphs, error bars indicate s.d., n =3. P values were determined with one-way ANOVA, using Tukey’s multiple comparisons test ( a , c ) or Student’s t -test ( d ). ** P <0.01. Full size image The control of superoxide by ARF in human melanocytes was also observed in a mouse context. Specifically, the levels of superoxide were three to five times higher in Arf −/− mouse embryonic fibroblasts (MEFs) retaining Trp53 expression than in Trp53 −/− MEFs retaining Arf expression ( Fig. 5d ), and these levels could be reduced by ectopic expression of Arf ( Supplementary Fig. 13 ). These data also suggested that p53, despite its role in senescence induced by mitochondrial dysfunction ( Supplementary Fig. 11 ), played no role in the mitochondrial function of Arf in the same cells. This was corroborated by experiments in human melanocytes and human epidermal fibroblasts treated with antimycin A, where efficient knockdown of p53 did not impair ARF-mediated control of superoxide ( Supplementary Fig. 14 ). Collectively, the above data suggest that ARF controls the production of superoxide from dysfunctional mitochondria in normal cells. We next extended our analysis of superoxide to a model with inducible depletion of BRAF E600 in ARF-expressing, TP53 -mutant melanoma cells ( Supplementary Fig. 15 ). Similar to the effects observed when glycolysis was inhibited in these cells ( Fig. 3a,b ), depletion of BRAF E600 caused a shift in metabolism towards oxidative phosphorylation [32] ( Supplementary Fig. 15 ). Interestingly, however, an increase in superoxide levels was observed only when the cells were depleted of ARF before the induction of the metabolic shift ( Fig. 5e and Supplementary Fig. 15c ). Hence, ARF was found to control superoxide production in all of our cellular models of mitochondrial dysfunction ( Fig. 5f ). ARF-mediated control of superoxide involves BCL-xL ARF has previously been associated with dissipation of ΔΨ m in the context of autophagy and apoptosis [10] . The pro-apoptotic activity of mitochondrial ARF was shown to depend on binding to the mitochondrial protein p32 (also known as C1QBP, gC1qR or HABP) [38] , whereas its autophagy-inducing activity was shown to involve the displacement of Beclin 1 from BCL-xL complexes through direct binding of ARF to BCL-xL [27] . In our melanocyte model of replicative senescence, dissipation of ΔΨ m was observed also in fully viable pre-senescent and senescent cells, and we found no evidence of any role of apoptosis-associated p32 or autophagy-associated Beclin 1. Specifically, the ARF RR98,99LS mutant, which is unable to interact with p32 (ref. 38 ), was as active as wild-type ARF in controlling superoxide production, and depletion of p32 had no effect on ARF-mediated control of superoxide levels ( Supplementary Fig. 16 ). Also, depletion of Beclin 1 had no effect on ARF activity, even though autophagy was clearly abrogated in melanocytes jointly depleted of Beclin 1 and BCL-xL, as seen by a reduced number of LC3 foci compared with melanocytes only depleted of BCL-xL ( Fig. 6a and Supplementary Fig. 16 ). 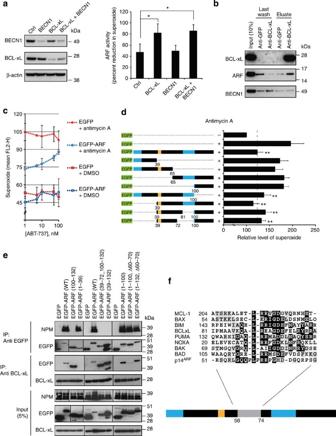Figure 6: ARF-mediated control of superoxide involves interaction with BCL-xL via a short acidic motif. (a) Control of superoxide by ARF following knockdown of BCL-xL, Beclin 1 or both. Left, immunoblot analysis showing knockdown efficiency. Right, percent reduction in superoxide levels achieved by pEGFP-ARF with or without knockdown of Beclin 1 and/or BCL-xL. (b) Co-immunoprecipitation of BCL-xL and ARF from mitochondria-enriched extracts from pre-senescent melanocytes. (c) Superoxide control by ARF is reversed by the BH3-mimetic BCL-xL inhibitor ABT-737. Nanomolar concentrations of ABT-737 were administered with DMSO or antimycin A (5 μM) to melanocytes transfected with a pEGFP control vector or pEGFP-ARF. (d) Left, diagrams depicting the various ARF deletion constructs. Domains conferring nucleolar localization and binding to nuclear interaction partners are shown in blue and the mitochondrial localization signal is shown in orange. Right, MitoSOX Red analysis showing the ability of each construct to down-regulate superoxide in normal melanocytes treated with antimycin A. The level of MitoSOX Red in EGFP-expressing cells is set at 100%. The stippled line indicates the MitoSOX Red level in antimycin A-treated cells transfected with pEGFP-ARF. (e) Co-immunoprecipitation of NPM, BCL-xL and ARF. U2OS cells were transfected with the indicated pEGFP-ARF expression constructs (d). Nuclear extracts were subjected to immunoprecipitation with EGFP antibodies and immunoblot analysis using anti-NPM and anti-EGFP antibodies. Cytoplasmic extracts were subjected to immunoprecipitation with anti-BCL-xL antibodies and immunoblot analysis using anti-BCL-xL and anti-EGFP antibodies. Shown are the input of NPM in nuclear extracts and the inputs of EGFP and BCL-xL in cytoplasmic extracts. (f) Alignment of residues 51–74 of human ARF with BH3 domains from BCL-2 family proteins. The diagram below depicts the relative localization of this region in wild-type ARF (shown in grey). In all graphs, error bars indicate s.d.,n=3.Pvalues were determined with one-way ANOVA, using Tukey’s multiple comparisons test. *P<0.05; **P<0.01. Figure 6: ARF-mediated control of superoxide involves interaction with BCL-xL via a short acidic motif. ( a ) Control of superoxide by ARF following knockdown of BCL-xL, Beclin 1 or both. Left, immunoblot analysis showing knockdown efficiency. Right, percent reduction in superoxide levels achieved by pEGFP-ARF with or without knockdown of Beclin 1 and/or BCL-xL. ( b ) Co-immunoprecipitation of BCL-xL and ARF from mitochondria-enriched extracts from pre-senescent melanocytes. ( c ) Superoxide control by ARF is reversed by the BH3-mimetic BCL-xL inhibitor ABT-737. Nanomolar concentrations of ABT-737 were administered with DMSO or antimycin A (5 μM) to melanocytes transfected with a pEGFP control vector or pEGFP-ARF. ( d ) Left, diagrams depicting the various ARF deletion constructs. Domains conferring nucleolar localization and binding to nuclear interaction partners are shown in blue and the mitochondrial localization signal is shown in orange. Right, MitoSOX Red analysis showing the ability of each construct to down-regulate superoxide in normal melanocytes treated with antimycin A. The level of MitoSOX Red in EGFP-expressing cells is set at 100%. The stippled line indicates the MitoSOX Red level in antimycin A-treated cells transfected with pEGFP-ARF. ( e ) Co-immunoprecipitation of NPM, BCL-xL and ARF. U2OS cells were transfected with the indicated pEGFP-ARF expression constructs ( d ). Nuclear extracts were subjected to immunoprecipitation with EGFP antibodies and immunoblot analysis using anti-NPM and anti-EGFP antibodies. Cytoplasmic extracts were subjected to immunoprecipitation with anti-BCL-xL antibodies and immunoblot analysis using anti-BCL-xL and anti-EGFP antibodies. Shown are the input of NPM in nuclear extracts and the inputs of EGFP and BCL-xL in cytoplasmic extracts. ( f ) Alignment of residues 51–74 of human ARF with BH3 domains from BCL-2 family proteins. The diagram below depicts the relative localization of this region in wild-type ARF (shown in grey). In all graphs, error bars indicate s.d., n =3. P values were determined with one-way ANOVA, using Tukey’s multiple comparisons test. * P <0.05; ** P <0.01. Full size image Although we observed no role of the BCL-xL-binding partner Beclin 1, depletion of BCL-xL caused a significant increase in the mitochondrial activity of ARF ( Fig. 6a ). We therefore considered whether BCL-xL is part of the mechanism by which ARF controls superoxide. This notion was corroborated by the fact that endogenous BCL-xL and ARF could be co-immunoprecipitated from mitochondria-enriched extracts from pre-senescent melanocytes ( Fig. 6b ). Furthermore, while the overexpression of ARF reduced superoxide levels in melanocytes treated with antimycin A, a chemical inhibitor of BCL-xL, ABT-737 (ref. 39 ), counteracted this effect at nanomolar concentrations and caused a dose-dependent restoration of superoxide levels ( Fig. 6c ). Apart from its canonical role in suppressing apoptosis by sequestering pro-apoptotic BCL-2 family proteins, BCL-xL has been shown to fulfil a role in mitochondrial homeostasis as a means to stabilize ΔΨ m (refs 40 , 41 , 42 ). The above findings are consistent with a model in which direct binding between ARF and BCL-xL disrupts the homeostatic activity of BCL-xL, leading to dissipation of ΔΨ m . Depolarization has been shown to be associated with a faster rate of electron transfer and may constitute a signal for elimination of individual mitochondria through mitophagy, two processes that would both serve to reduce the production of superoxide. To address whether the ability of ARF to control superoxide was dependent on mitophagy, we examined Parkin, a marker of early mitophagy. Consistent with findings in other cell types [43] , inhibition of oxidative phoshorylation by antimycin A triggered translocation of Parkin to mitochondria ( Supplementary Fig. 17 ). Furthermore, depletion of Parkin led to an increase in superoxide levels (data not shown). However, the reduction in Parkin levels did not significantly rescue the superoxide-controlling effect of ARF, and loss of mtDNA copy number and mitochondrial proteins did not occur within the first 90 min of antimycin A treatment when a significant reduction in superoxide had already occurred ( Supplementary Fig. 17 ). These data suggest that mitophagy could be a late effect of the response of ARF to mitochondrial dysfunction. A short acidic motif in ARF interacts with BCL-xL ARF shows little homology with other proteins [1] and only few functional domains have been identified, including a region required for binding to nuclear interaction partners such as NPM and HDM2 (residues 1–14) [44] , [45] , [46] , [47] , a mitochondrial import signal (residues 41–46) [48] and a region involved in nucleolar import (residues 82–101) [49] . The latter region has also been reported to be a binding site for the mitochondrial protein p32 (ref. 38 ). The site of interaction with BCL-xL has remained unknown. To map the functional domain(s) involved in the control of mitochondrial superoxide production, we analysed a series of enhanced green fluorescent protein (EGFP)-tagged ARF deletion constructs ( Fig. 6d ) in melanocytes treated with antimycin A. In parallel, we investigated the ability of these constructs to interact with endogenous BCL-xL and NPM after overexpression in U2OS cells. These cells express high endogenous levels of both proteins and have been extensively used for identifying ARF-interaction partners. The deletion analysis showed that ARF can maintain low levels of superoxide independent of its known nuclear binding and localization domains ( Fig. 6d ). Specifically, a protein composed of residues 39–72 and 100–132 (ARF 39–72_100–132 ) did not co-immunoprecipitate with NPM ( Fig. 6e ) and predominantly localized outside the nucleus in U2OS cells and melanocytes ( Supplementary Fig. 18 ), yet was as active as full-length ARF in the superoxide analysis ( Fig. 6d ) and retained the ability to co-immunoprecipitate with BCL-xL ( Fig. 6e ). Furthermore, ARF 1–100 and ARF 100–132 both co-immunoprecipitated with BCL-xL, consistent with the presence of at least two separate binding sites for BCL-xL, including one located in the very carboxyl-terminal (C-terminal) part of ARF. Interestingly, ARF 1–100 and ARF 39–72_100–132 were equally active in controlling superoxide production ( Fig. 6d ) and both co-immunoprecipitated with BCL-xL ( Fig. 6e ), suggesting that the ability of ARF to control superoxide and the ability to interact with BCL-xL map to the same region shared by these proteins (residues 39–72). Alignment of ARF proteins from different species revealed that this region contains an invariably conserved sequence motif, G(H/D)DDGQ (residues 65–70; Supplementary Fig. 19 ). Interestingly, the two aspartates, D67 and D68, represent two of only three negatively charged residues in the entire ARF protein. Another unusual feature of this motif was a weak resemblance to the GDE/D motif found in BH3 domains of BCL-2 family proteins, where two adjacent negatively charged amino acids are required for interaction with positively charged residues within the binding pocket of anti-apoptotic BCL-2 proteins [50] . This observation prompted us to perform alignments between this region in ARF and known BH3 domains in a range of BCL-2 family proteins. As shown in Fig. 6f , there were a number of similarities between ARF and known BH3 domains, including highly conserved glycine, arginine and leucine residues. However, this region in ARF is not a bona fide BH3 domain, as it contains four prolines (residues 59, 61, 64 and 72), which would prevent the adaptation of an α-helical structure. Nevertheless, when the core of this region (residues 60–70) was deleted, the interaction of ARF 1–100 with BCL-xL was abolished, confirming that it acts as a BCL-xL-binding site ( Fig. 6e ). Melanoma-predisposing ARF mutations affect the GHDDGQ motif Intracellular production of ROS increases the risk of cancer-promoting mutations. A variety of cellular mechanisms have evolved to protect against ROS, often involving the ‘care-taker’ class of tumour suppressors [51] . Having shown that ARF limits the proliferative capacity of melanocytic cells with dysfunctional mitochondria and limits superoxide production, we asked if melanoma-predisposing CDKN2A mutations affected these functions. Indeed, among 23 germline CDKN2A mutations introducing amino acid substitutions in ARF (refs 14 , 19 , 52 ), eight affected residues 56–74, suggesting a non-random distribution. In contrast, reported mutations associated with sporadic melanoma did not cluster within this region ( Fig. 7a ). Among the germline mutations, six of the missense mutations affected the five evolutionarily conserved residues within the acidic motif ( Fig. 5a ; χ 2 -test, P =4 × 10 −8 ), including D68H, the second most common CDKN2A mutation associated with familial melanoma [14] and three mutations affecting glycine 65 (refs 14 , 19 ) ( Fig. 7b ). 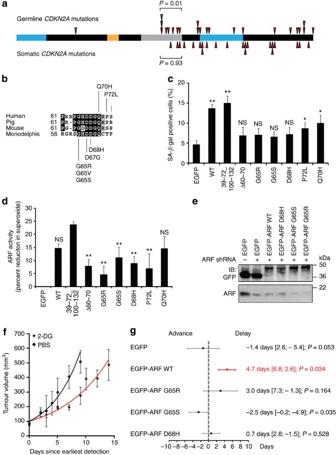Figure 7: Germline mutations inCDKN2Acluster to a short acidic motif in ARF and affects melanoma growth. (a) Spectra of somatic and germlineCDKN2Amissense mutations associated with melanoma. Mutations specific for ARF are indicated by green triangles; mutations affecting both ARF and p16 are indicated by red triangles. The germlineCDKN2Amutations have been reported by GenoMEL study centres14,19,52. Information on somaticCDKN2Amutations in melanoma was obtained from COSMIC (http://www.sanger.ac.uk/cosmic; accessed September 2011)64.Pvalues were determined usingχ2-tests. (b) Shown is a diagram of evolutionarily conserved residues in the vicinity of the short acidic motif in ARF and germlineCDKN2Amutations affecting these residues. (c,d) SA-β-gal staining (c) and superoxide levels (d) in ARF-negative FM3 melanoma cells following transfection with pEGFP or pEGFP-ARF constructs harbouring the indicated deletions or point mutations. Ind, the level of superoxide was calculated relative to the level found after pEGFP transfection to provide a measure of the percent reduction in superoxide exerted by each ARF construct. Error bars (c,d) indicate s.e.m.,n=3.Pvalues were determined with one-way ANOVA, using Tukey’s multiple comparisons test.Post hoctests are shown relative to EGFP (c) or relative to the most active ARF construct (d). NS, not significant; *P<0.05; **P<0.01. (e) Immunoblot analysis showing residual level of endogenous ARF in p53-mutated FM55-M2 melanoma cells after stable knockdown of ARF and overexpression of EGFP, EGFP-ARF (wild type, WT) or EGFP-ARF harbouring the indicated point mutations. (f) Effect of 2-DG on thein vivogrowth of FM55-M2 cells overexpressing EGFP-ARF (WT) and depleted of endogenous ARF. Error bars indicate s.d.,n=7 (2-DG),n=8 (PBS). (g) Mean growth-delaying effect of 2-DG on FM55-M2 xenografts in NOG mice. The cells were depleted of endogenous ARF and transfected with EGFP, EGFP-ARF or EGFP-ARF harbouring the indicated point mutations. Responses to 2-DG are shown as an advance (left side) or delay (right side) in the time required for the tumours to grow from the earliest detection (100 mm3) to a volume of 500 mm3. Error bars indicate 95% confidence intervals.Pvalues were determined by Student’st-test. Figure 7: Germline mutations in CDKN2A cluster to a short acidic motif in ARF and affects melanoma growth. ( a ) Spectra of somatic and germline CDKN2A missense mutations associated with melanoma. Mutations specific for ARF are indicated by green triangles; mutations affecting both ARF and p16 are indicated by red triangles. The germline CDKN2A mutations have been reported by GenoMEL study centres [14] , [19] , [52] . Information on somatic CDKN2A mutations in melanoma was obtained from COSMIC ( http://www.sanger.ac.uk/cosmic ; accessed September 2011) [64] . P values were determined using χ 2 -tests. ( b ) Shown is a diagram of evolutionarily conserved residues in the vicinity of the short acidic motif in ARF and germline CDKN2A mutations affecting these residues. ( c , d ) SA- β -gal staining ( c ) and superoxide levels ( d ) in ARF-negative FM3 melanoma cells following transfection with pEGFP or pEGFP-ARF constructs harbouring the indicated deletions or point mutations. In d , the level of superoxide was calculated relative to the level found after pEGFP transfection to provide a measure of the percent reduction in superoxide exerted by each ARF construct. Error bars ( c , d ) indicate s.e.m., n =3. P values were determined with one-way ANOVA, using Tukey’s multiple comparisons test. Post hoc tests are shown relative to EGFP ( c ) or relative to the most active ARF construct ( d ). NS, not significant; * P <0.05; ** P <0.01. ( e ) Immunoblot analysis showing residual level of endogenous ARF in p53-mutated FM55-M2 melanoma cells after stable knockdown of ARF and overexpression of EGFP, EGFP-ARF (wild type, WT) or EGFP-ARF harbouring the indicated point mutations. ( f ) Effect of 2-DG on the in vivo growth of FM55-M2 cells overexpressing EGFP-ARF (WT) and depleted of endogenous ARF. Error bars indicate s.d., n =7 (2-DG), n =8 (PBS). ( g ) Mean growth-delaying effect of 2-DG on FM55-M2 xenografts in NOG mice. The cells were depleted of endogenous ARF and transfected with EGFP, EGFP-ARF or EGFP-ARF harbouring the indicated point mutations. Responses to 2-DG are shown as an advance (left side) or delay (right side) in the time required for the tumours to grow from the earliest detection (100 mm 3 ) to a volume of 500 mm 3 . Error bars indicate 95% confidence intervals. P values were determined by Student’s t -test. Full size image To examine the possible functional consequences of these mutations, we generated EGFP-tagged ARF constructs harbouring individual mutations (G65R, G65S, D68H, Q70H and P72L). These constructs were then tested for their ability to induce senescence and reduce superoxide production in melanoma cells with a p53-proficient/ARF-deficient background. All of these mutations reduced the activity of ARF with respect to senescence ( Fig. 7c ) and superoxide ( Fig. 7d ), with G65R, G65S and D68H reaching statistical significance on both endpoints (analysis of variance (ANOVA), P <0.05). As shown in Supplementary Figs 13a and 18 , overexpressed ARF accumulated in the nucleus of melanocytic cells, with potential confounding effects on cell growth exerted via its canonical p53-dependent function. Furthermore, as the mitochondrial activity of ARF is masked in melanomas due to the glycolytic phenotype of these cells with little dependence on oxidative phosphorylation ( Fig. 3 ), we investigated the function of ARF in p53-mutated melanoma cells in response to inhibition of glycolysis. As shown in Figs 3c and 5e , ARF translocated to mitochondria and controlled superoxide production in response to the metabolic shift. Also, the growth of these cells was severely inhibited by 2-DG [32] , which was partially rescued by the depletion of endogenous ARF ( Supplementary Fig. 20a ). Transfection of melanoma cells with EGFP-ARF constructs in a background of endogenous ARF depletion ( Fig. 7e ) suggested that growth in the presence of 2-DG was suppressed via ARF, and that the mutant forms of ARF had lost this growth-suppressive activity ( Supplementary Fig. 20b ). Most importantly, the metabolism-dependent growth suppression could also be observed in vivo , when the same cells were injected into NOG mice followed by three-weekly injections of 2-DG. While 2-DG caused a significant growth delay of tumours overexpressing wild-type ARF (4.7 days; 95%CI: 2.6–6.8; P =0.034), no such delay was observed for tumours expressing mutant ARF proteins ( Fig. 7f,g ). Interaction between BCL-xL and the F1 β subunit of the F 1 F O ATP synthase is important for upholding ΔΨ m (refs 41 , 42 ). Immunoprecipitation experiments confirmed weak associations between BCL-xL and the F 1 F O ATP synthase subunits α and β and inhibitory factor 1 in mitochondrial extracts from ARF-expressing melanoma cells. When these cells were treated with 2-DG to force usage of their dysfunctional mitochondria, the interaction of BCL-xL with the F 1 F O ATP synthase subunits was no longer detectable ( Fig. 8a ). In contrast, 2-DG caused an increased association between BCL-xL and F 1 F O ATP synthase subunits in ARF-depleted melanoma cells, which could be prevented by the addition of exogenous ARF to the immunoprecipations ( Fig. 8b ). 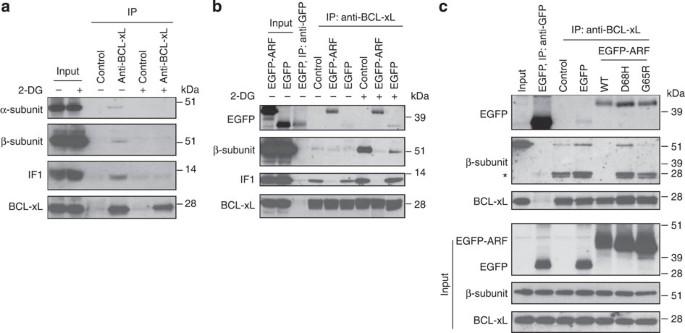Figure 8: Acidic motif mutations affect the ability of ARF to disrupt the interaction between BCL-xL and the F1FOATP synthase. (a) Immunoprecipitation (IP) of BCL-xL from mitochondrial extracts from FM55-M2 melanoma cells in the presence or absence of 20 mM 2-DG. Precipitates were investigated for BCL-xL and the F1 subunits α and β and inhibitory factor 1 (IF1). (b) IP of BCL-xL from mitochondrial extracts from ARF-depleted FM55-M2 cells in the presence or absence of 20 mM 2-DG. Purified EGFP-ARF or EGFP proteins were added to the IPs. Precipitates were investigated for EGFP, BCL-xL, the F1 subunit β and IF1. (c) IP of BCL-xL from mitochondrial extracts from ARF-depleted FM55-M2 cells in the presence of 2-DG. EGFP, EGFP-ARFWT, EGFP-ARFD68Hor EGFP-ARFG65Rwere added to the IPs. Precipitates were investigated for EGFP, BCL-xL and the F1 subunit β. A degradation product of subunit β is marked with an asterisk. Figure 8: Acidic motif mutations affect the ability of ARF to disrupt the interaction between BCL-xL and the F 1 F O ATP synthase. ( a ) Immunoprecipitation (IP) of BCL-xL from mitochondrial extracts from FM55-M2 melanoma cells in the presence or absence of 20 mM 2-DG. Precipitates were investigated for BCL-xL and the F1 subunits α and β and inhibitory factor 1 (IF1). ( b ) IP of BCL-xL from mitochondrial extracts from ARF-depleted FM55-M2 cells in the presence or absence of 20 mM 2-DG. Purified EGFP-ARF or EGFP proteins were added to the IPs. Precipitates were investigated for EGFP, BCL-xL, the F1 subunit β and IF1. ( c ) IP of BCL-xL from mitochondrial extracts from ARF-depleted FM55-M2 cells in the presence of 2-DG. EGFP, EGFP-ARF WT , EGFP-ARF D68H or EGFP-ARF G65R were added to the IPs. Precipitates were investigated for EGFP, BCL-xL and the F1 subunit β. A degradation product of subunit β is marked with an asterisk. Full size image Consistent with the existence of two BCL-xL-binding sites in ARF, the D68H and G65R mutations both reduced, but did not abrogate, the interaction between BCL-xL and ARF ( Supplementary Fig. 21 ). Furthermore, unlike ARF WT , ARF D68H and ARF G65R did not disrupt the interaction between BCL-xL and the F1 β subunit of the F 1 F O ATP synthase, even when the mutant proteins were added to the anti-BCL-xL immunoprecipitations in higher amounts than the corresponding wild-type protein ( Fig. 8c ). Collectively, these data suggest that germline mutations targeting the small acidic motif in ARF affect the interaction between ARF and BCL-xL by reducing the overall affinity of ARF for BCL-xL or impairing the ability of ARF to disrupt the interaction between BCL-xL and the F 1 F O ATP synthase. Several studies have shown that ARF can localize to mitochondria when overexpressed in transformed cells, and a number of mitochondrial interaction partners for ARF have been identified [10] , [27] , [38] , [53] . In various cellular model systems, ARF interacts with p32 and induces mitochondrial membrane depolarization, leading to apoptotic or autophagic cell death responses [38] , [54] . Small fractions of endogenous ARF have been demonstrated in mitochondrial preparations from MEFs and human tumour cells [55] ; however, the functional significance of endogenous mitochondrial ARF has not been determined, partly because cellular signals or mechanisms that could trigger translocation of ARF to mitochondria have remained elusive. Our investigation of ARF in the melanocytic lineage was prompted by previous work implicating ARF-specific CDKN2A germline mutations in melanoma susceptibility [14] , [15] , [16] , [17] , [18] , [19] . Our data show that endogenous ARF is constitutively expressed as a cytoplasmic protein in melanocytes and is recruited to injured or dysfunctional mitochondria to induce loss of membrane potential and maintain low steady-state levels of intracellular superoxide. This mechanism could be activated by pharmacological inhibition of oxidative phosphorylation in normal melanocytes, as well as in melanoma cells undergoing a metabolic shift in response to inhibition of glycolysis. ARF was fully capable of controlling superoxide production in cells depleted of p32 or p53 and after deletion of the domains required for interaction with p32 and MDM2, suggesting the involvement of a mechanism that is different from the known autophagic and p53-dependent functions of ARF. In our models involving induced mitochondrial dysfunction, we cannot exclude that part of the ARF-mediated reduction in superoxide levels could be due to loss of mitochondrial mass by Parkin-mediated mitophagy, as has been demonstrated in other models using chemical inhibitors of the electron transport chain [43] . Nevertheless, under standard cell culture (stressful) conditions where mitochondrial dysfunction evolves progressively, the fraction of mitochondrial ARF increased with replicative age without any significant reduction in the number of mitochondria, suggesting that ARF can translocate to mitochondria and act in a more subtle way to control superoxide production without inducing mitophagy. Indeed, the severely reduced RCR in pre-senescent cells could be rescued by depletion of ARF, consistent with an overall change in polarization across the mitochondrial inner membrane rather than a change in the number of mitochondria. The effect of ARF on superoxide production may be directly related to its ability to lower ΔΨ m , similar to the mechanism by which chemical uncouplers diminish superoxide production by dissipating the proton gradient. In our study, we have demonstrated a physical interaction between endogenous ARF and BCL-xL in pre-senescent melanocytes and shown that control of superoxide by ARF involves BCL-xL. Apart from its canonical anti-apoptotic function associated with balancing out pro-apoptotic BCL-2 family proteins, BCL-xL has been shown to affect VDAC and the F 1 F O ATP synthase to maintain mitochondrial homeostasis [40] , [41] , [42] . In primary neurons, a cell type that shares many developmental, physiological and molecular properties with melanocytes, BCL-xL stabilizes the mitochondrial membrane potential, and BCL-xL-overexpressing cells have a greater, yet, underutilized energetic capacity as judged from increased oxygen consumption over basal levels under depolarizing conditions [41] . Our results are consistent with a function of ARF as an inhibitor of BCL-xL, as high expression of ARF in pre-senescent cells was associated with lower energetic capacity (hypopolarization and low RCR levels), while depletion of ARF conferred a higher energetic capacity (hyperpolarization and increased RCR levels). Furthermore, immunoprecipitation of BCL-xL in the presence of ARF confirmed that ARF inhibits interactions between BCL-xL and the F 1 F O ATP synthase. These data suggest that BCL-xL and ARF, apart from their opposing roles in autophagy/apoptosis, have evolved as opposing components in the regulation of the energetic capacity of oxidative phosphorylation in fully viable cells. We propose that in the context of its ability to control superoxide levels, ARF can be regarded as a cell-protective mechanism that guards against mitochondrial dysfunction. ARF is an unusual protein based on biochemical criteria, being unstructured and highly basic (pI>12), and showing no strong homology with other proteins [1] . The ability of ARF to control superoxide production from dysfunctional mitochondria was mapped to an evolutionarily conserved motif, GHDDGQ (residues 65–70), which contains two of only three acidic amino acids present in human ARF. Mechanistically, this region in ARF was shown to interact with BCL-xL, and the superoxide-controlling activity of ARF was abolished by the BCL-xL antagonist ABT-737 and by melanoma-predisposing mutations affecting single residues within the GHDDGQ motif. Most important, mutations affecting the negative charge of this motif, for example, G65R and D68H, abolished the ability of ARF to disrupt the binding between BCL-xL and the F 1 F O ATP synthase. On the basis of the primary sequence of the short acidic motif and its surrounding region, structural comparison analysis revealed similarities with BH3 domains of BCL-2 family proteins. However, the presence of four prolines in the surrounding sequence would prevent the formation of the α-helical structure characteristic of canonical BH3 domains. The presence of prolines in BH3-like domains of proteins that can interact with anti-apoptotic proteins is not without precedence. For example, the pro-apoptotic activity of Atg12 depends on a BH3-like domain that contains a single proline, preventing the formation of an α-helical structure but still enabling binding into the hydrophobic cleft of BCL-2 (ref. 56 ). Another similarity we found between ARF and BCL-xL-interacting BH3-only proteins was a second BCL-xL-binding site in the C terminus. This region in ARF comprises an evolutionary conserved sequence important for mitochondrial localization of ARF, but consistent with the presence of two BCL-xL-binding sites, mutations in this region were unable to abrogate the interaction between ARF and BCL-xL [53] . The cytoplasmic localization of ARF in primary melanocytes raises the question of whether ARF-associated melanoma susceptibility may be attributed to the function of ARF described here, that is, the ability to control the formation of ROS from injured or dysfunctional mitochondria. It is well established that uncontrolled ROS production stimulates tumour formation through the oxidation of DNA and subsequent mutation of oncogenic drivers. As a reduction in the levels of ARF in normal human melanocytes generates a high membrane potential and an increased production of superoxide, monoallelic loss of ARF function in mutation carriers may increase melanoma risk indirectly through an increased mutation rate. Melanoma has the highest prevalence of somatic mutations among human cancers [57] , which has in part been attributed to exposure to ultraviolet light. Interestingly, however, another characteristic of the mutation pattern in melanoma is a high proportion of C>A/G>T transversions occurring in a distinctive sequence context [58] , which is consistent with ROS-induced damage to guanine [59] and thus could be a result of ARF loss. Oncogene-induced senescence (OIS) is a cell-autonomous mechanism that induces irreversible arrest of potentially tumorigenic cells. Previous studies have identified the ‘gate-keeper’ function of p16 as an important component of OIS in melanocytes [23] , which can be upregulated in response to oncogenic BRAF or NRAS. A similar role of ARF in OIS has not been found, and a subset of melanomas can progress despite the expression of cytoplasmic ARF. Our data show that this apparent paradox should probably be viewed in the context of the fundamental changes in metabolism that occur during melanoma development. Mutated BRAF, when acting as an early melanoma driver, promotes metabolic reprogramming by suppressing oxidative phosphorylation and promoting glycolysis [32] , [33] . Consistent with a ‘watching and waiting’ function of ARF, its growth-inhibitory function was inactive in BRAF V600E /ARF-expressing melanoma cells, but could be induced in vitro and in vivo by redirecting the metabolism toward mitochondrial oxidative metabolism. This is, to our knowledge, the first example of how the normal function of a tumour suppressor can be reactivated and studied in transformed cells by reverting the metabolic state towards that present in the normal counterpart cells. In conclusion, we have identified a cell-protective mechanism of ARF in melanocytes that is targeted in familial melanoma. Our data fit into a conceptual framework in which proteins guarding against mitochondrial dysfunction can serve as tumour-suppressive barriers, whereas oncogenes can help cells evading such barriers by redirecting cellular metabolism. Cells and reagents Human epidermal neonatal melanocytes (batches 4C0197, 4C0340, 5C0272 and 200708522) and human dermal neonatal fibroblasts were purchased from Invitrogen. The fibroblasts were used for experiments within the first 10 passages. U2OS cells were obtained from ATCC. FM3 and FM55-M2 melanoma cells were generated in our laboratory [60] . Information on antibodies is presented in Supplementary Table 1 . Mitotracker Red (CM-H 2 XROS), MitoSOX Red and Carboxy-H 2 DCFDA (Image-iT) were purchased from Invitrogen. Oligomycin A, antimycin A, 3,3′-dihexyloxacarbocyanine iodide (DiOC 6 (3)) and carbonyl cyanide 3-chlorophenylhydrazone (CCCP) were purchased from Sigma-Aldrich. Cell culture and generation of ARF/p16-depleted melanocytes Melanocytes were routinely cultured in Medium 254 and Human Melanocyte Growth Supplement (Invitrogen) at 37 °C and 5% CO 2 . To generate the stable knockdown of ARF and p16, we used pSuper plasmids containing resistance to G418 (refs 61 , 62 ). Stable melanocytic transfectants were selected using increasing concentrations of G418 (Invitrogen) diluted in conditioned medium from young melanocytes (100–1,000 μg ml −1 during a period of 6 weeks) in the presence of stem cell factor (100 ng ml −1 , Stratmann Biotech) and endothelin-1 (10 ng ml −1 , Sigma-Aldrich). The medium was changed three times a week. To obtain cultures that grew beyond the first passage, both ARF and p16 had to be efficiently reduced. Two independent cultures were made. HEM-1 was made by pooling 28 large G418-resistant colonies 6 weeks after transfection with pSuper expressing shRNA to a target sequence within CDKN2A exon 2 (p16/ARF-exon 2, Supplementary Table 1 ). HEM-2 was made from a single G418-resistant clone transfected with pSuper expressing shRNA to a target within CDKN2A exon 1α (p16-exon1, Supplementary Table 1 ), which could be further propagated due to a spontaneous loss of ARF. Immunocytochemistry Cells (10 4 ) were placed on glass cover slips in droplets of complete growth medium. Once adherent, the cover slips were covered with growth medium and incubated. When indicated, cells were treated with 200 nM Mitotracker dye in growth medium for 30 min before fixation. For immunofluorescence analysis, we used the Zeiss LSM510 system, combining laser scanning and fluorescent microscope. Images were acquired and processed using the ZEN software (Zeiss). mtDNA detection using 4′,6-diamidino-2-phenylindole was achieved by reducing the interfering nuclear DNA signal by laser bleaching, using the diode laser (405 nm) at maximum power for 5–10 min. For SR-SIM, samples were examined on a Zeiss Axioimager Z.1 platform equipped with the Elyra PS.1 super-resolution system using Zeiss Alpha Plan Apochromat × 63/NA1.40 oil objectives (total magnification × 1,008) with oil (Immersol 518F, Zeiss). Light source for SR-SIM included diode lasers (405, 488 and 568 nm). Images were captured with an EM-CCD camera (Andor iXON EM+; 1,004 × 1,002 px, cooled at −64 °C, 16-bit). Up to seven 110-nm Z-stacks were acquired per image. Acquisition and image processing was done using Zeiss Zen 11 software (Zen Blue version, Carl Zeiss Microscopy, Jena). Flow cytometric analysis of ΔΨm Age-associated changes in mitochondrial membrane potential were determined by flow cytometry. Adherent cells were stained with 25 nM DiOC 6 (3) for 20 min in the tissue culture incubator. Alternatively, ΔΨ m was measured using the MitoProbe JC-1 Assay Kit (Invitrogen). Samples were analysed in a FACSort cytometer (Becton Dickinson). Results were based on mean fluorescence in the FL1 channel in the case of DiOC 6 (3) or dot blots of FL2-H versus FL1-H in the case of JC-1. ATP measurements The concentration of ATP was determined using a modified method based on the ATPlite luminescence assay system (Perkin Elmer). The modification involved seeding 2.5 × 10 5 cells in 5-cm dishes the day before, collecting samples by lysing the cells with 750 μl of lysis solution (2:1 melanocyte medium: cell lysis buffer (ATPlite, Perkin Elmer)) and immediately freezing the samples in liquid nitrogen. Triplicate samples were made for each measurement. Cell number and diameter were recorded in parallel using a Z2 Coulter particle and cell counter (Beckman Coulter), based on triplicate samples. As a standard, a serial dilution of ATP was prepared in lysis solution and stored frozen for the same length of time as the samples. ATP concentrations were measured based on triplicate 150-μl aliquots taken from each frozen sample, each mixed with 50 μl of substrate solution and loaded onto white-walled 96-well plates. Luminescence was recorded in a Fluostar Omega microplate reader (BMG Labtech). Flow cytometric analysis of ROS and superoxide General ROS levels were detected using carboxy-H 2 DCFDA and superoxide was detected using MitoSOX Red according to the manufacturer’s instructions. MitoSOX Red (5 μM) or Carboxy-H 2 DCFDA (25 μM) combined with propidium iodide (10 μg ml −1 ) were loaded onto the cells for 30 and 40 min, respectively. When combined with cell transfections, fluorescence-activated cell sorting analysis was performed 24 h post transfection by gating for GFP-positive cells and measuring mean MitoSOX Red stain in the FL2 channel. As indicated in the text, transfections were performed with various EGFP-ARF constructs or pX, pX: ARF or pX: myc-p16 plasmids combined in a 9:1 ratio with pMaxGFP plasmid (Amaxa). In fibroblasts, transfections were first made with pSuper-p53sh or empty pSuper vector. The next day, cells were transfected with pX or pX:p14ARF (in a 9:1 ratio with pMaxGFP), and treatment with antimycin A (1 μM) commenced the day after. MitoSOX Red staining was measured by fluorescence-activated cell sorting analysis in cells treated for 1 h with antimycin A. Senescence, apoptosis and necrosis Senescent cells were detected by staining for SA- β -Gal activity, and apoptotic and necrotic cells were detected using Hoechst/Sytox staining, as previously described [61] . mtDNA copy number DNA was isolated from melanocytes using the QIAamp DNA Mini Kit (Qiagen). PCR was performed in a Roche LightCycler 2.0 using the FastStart DNA Master PLUS SYBR Green I Kit (Roche) and previously described primers [63] . Real-time quantitative PCR Total RNA was isolated using the NucleoSpin RNA II Kit (Macherey-Nagel). Reverse transcription was performed using the SuperScript III reverse transcriptase (Invitrogen). Real-time PCR was performed using the Roche LightCycler 2.0 and the FastStart DNA Master PLUS SYBR Green I. Primer sequences are listed in Supplementary Table 3 . Transfection and RNA interference Transfection of melanocytes was performed using the Amaxa nucleofection technology. Programmes for transfection of melanocytes were as recommended by the manufacturer. We routinely obtained a transfection efficiency of at least 50%. Transient RNA interference was performed using a 1 μM mixture of two synthetic siRNAs to ARF (2 μM in the case of pre-senescent melanocytes) ( Supplementary Table 2 ), or SMARTpools of siRNAs to p53, Parkin, p32, Beclin 1 or BCL-xL (Dharmacon). FM3 and FM55-M2 cells were transfected using LipofectAMINE 2000 (Invitrogen), either once for superoxide analysis or twice for analysis of senescence (FM3) or generation of stable cell lines (FM55-M2). Following the second transfection, cells were selected using 500 μg ml −1 G418 or 1 μg ml −1 puromycin for up to 10 days. Generation of stable and inducible FM55-M2 cell lines The FM55-M2: TREx: V600E BRAF sh cell line has been previously described [32] . To generate stable ARF- and p16-depleted versions of this cell line, the tetracycline-responsive H1-promoter present in pSuperior/Puro R was replaced by expression cassettes containing non-inducible H1 promoter and shRNA-expressing inserts from pSuper/G418R constructs described above, making use of the EcoRI and HindIII sites in the cloning. The resulting pSuperior/PURO R : p16sh and pSuperior/PURO R : ARFsh expression constructs were used for transfection followed by puromycin selection as described above. The pSuperior/PURO R : ARFsh construct was also stably transfected into parental FM55-M2 cells and the resulting pool of ARF-depleted cells further transfected with EGFP, EGFP-ARF (wild type) or EGFP-ARF constructs harbouring mutations followed by G418-selection. Cell fractionation and immunoblotting Routine cytoplasmic and nuclear extracts were prepared using the NE-PER method (Pierce). When mitochondria were prepared as part of the procedure, we used a method described by Itahana and Zhang [38] , modified to include additional washes after the initial lysis with 0.015% digitonin and lysis of the digitonin-insoluble pellet with 0.2% Triton-X-100/hypotonic buffer on ice for 5 min. From the remaining material, nuclear extracts were prepared with hypertonic buffer (20 mM HEPES pH 7.4, 400 mM KCl, 2 mM MgCl 2 , 1 mM EDTA, 0.5% Triton-X-100, 10% glycerol). To detect ARF, proteins were separated on 12% NuPAGE gels using MES running buffer (Invitrogen). Membranes were incubated overnight with 2 μg ml −1 anti-ARF antibodies followed by 2 h of incubation at room temperature. HeLa cell extracts were used as an internal standard. When indicated in the text, quantification of protein expression was performed using the LAS-1000 luminescent image analyzer and Multi gauge V2.2 software (Fujifilm). Uncropped immunoblots blots are shown in Supplementary Fig. 22 . Immunoprecipitation U2OS cells (10 7 ) were transfected with each EGFP-ARF construct, left in the incubator for 8 h and subsequently extracted with 500 μl of hypotonic buffer containing 0.015% digitonin as described above. Following centrifugation, the pellet was extracted 10 min on ice with 100 μl of hypotonic buffer containing 0.135% digitonin, 0.015% NP-40 and 30% glycerol. The two extracts were mixed for immediate immunoprecipitation using anti-BCL-xL antibodies. The pellet after second centrifugation was extracted 10 min on ice with 100 μl of RIPA buffer, centrifugated and re-extracted 10 min on ice with 500 μl of hypotonic buffer containing 0.135% digitonin, 0.015% NP-40 and 30% glycerol. The two extracts were mixed for immediate immunoprecipitation using anti-EGFP antibodies. Immunoprecipitations were performed using Dynabeads (Invitrogen), which had previously been conjugated to rabbit or mouse antibodies using dimethyl pimelimidate. Each reaction included 2.5 × 10 7 beads (sheep-anti-rabbit) conjugated to a maximum of 2.5 μg rabbit antibodies and 2.5 × 10 7 beads (sheep-anti-mouse) conjugated to a maximum of 5 μg mouse antibodies. Information on antibodies is presented in Supplementary Table 1 . Co-immunoprecipitations of BCL-xL and F 1 F O ATP synthase subunits were performed from mitochondria-enriched fractions derived from parental or ARF-depleted FM55-M2 cells. EGFP, EGFP-ARF, EGFP-ARF(D68H) and EGFP-ARF(G65R) proteins were produced by transient transfection of expression constructs in U2OS followed by affinity-purification using anti-GFP beads. Increasing amounts of these proteins, a 1:1 mixture of beads coupled to rabbit and mouse anti-BCL-xL antibodies and mitochondria-enriched fractions were mixed for 1 h before adding a final concentration of 0.135% digitonin, 0,015% NP-40 and 5% glycerol. Immunoprecipitations were performed overnight at 4 °C, and a series of washing steps were conducted using a magnet and hypotonic buffer containing 0.135% digitonin, 0.015% NP-40, 5% glycerol and an increasing concentration of NaCl. Elution was performed using 0.1 M citric acid followed by neutralization with NaOH. EGFP-ARF constructs pShuttle-CMV vectors encoding wild-type ARF were kindly provided by Dr Yanping Zhang. The pShuttle-CMV-ARF plasmid was restricted with SmaI and XbaI and the released fragment encoding the C-terminal part of ARF was cloned into the same sites of pEGFP-C1 (Clontech) to generate the plasmid encoding ARF 100–132 . In addition, the pShuttle-CMV-ARF plasmid was digested with HindIII and BglII, and the ARF-encoding fragment was ligated into pEGFP-C1 digested with the same two enzymes, to generate the plasmid encoding wild-type ARF. The pEGFP(C1)-ARF plasmid was digested with XbaI, treated with Mung Bean nuclease, digested with SmaI and finally self-ligated to generate pEGFP-ARF 1–100 . Vectors (p3xFLAG-CMV; Sigma-Aldrich) encoding 3xFLAG-ARF(aa1–65) or 3xFLAG-ARF(aa65–132) were kindly provided by Dr Barbara Majello. The p3xFLAG-ARF(aa 1–65) and p3xFLAG-ARF(aa 65–132) vectors were digested with EcoRI and XbaI to release ARF-encoding fragments, which were then ligated into pEGFP-C1 digested with the same two enzymes to generate pEGFP-ARF 1–65 and pEGFP-ARF 65–132 , respectively. pEGFP-C2 (Clontech) expressing EGFP-ARF(aa 39–132) or EGFP-ARF(aa 1–39) were kindly provided by Dr Alessandra Pollice. The pEGFP-ARF(aa 39–132) plasmid was digested with BbsI and SmaI and then ligated onto synthetic fragments, which had appropriate overhangs for cloning into BbsI and SmaI sites and replaced parts of the ARF sequence between the two sites, yielding pEGFP-ARF 39–72_100–132 and pEGFP-ARF 39–81_100–132 . EGFP-ARF constructs containing point mutations or a deletion of residues 60–70 were generated by PCR site-directed mutagenesis using reagents and protocols provided with the Quickchange II kit (Agilent). See Fig. 6 for a schematic presentation of all constructs. Oxygen consumption and extracellular acidification Measurements of OCR and extracellular acidification rate (ECAR) in FM55-M2 cells were performed using the Seahorse XF24 analyzer (Seahorse Bioscience) as previously described [32] . Briefly, cells were seeded in XF24 V7 culture microplates at a density of 3.0 × 10 4 cells per well in growth medium (RPMI medium) a day before the experiment. OCR and ECAR were investigated in basic Dulbecco's modified Eagle's medium medium containing 5 mM glucose (pH 7.4). Oligomycin (1 μM) or 2-DG (10 mM) was added for inhibition of OCR or ECAR, respectively. Melanocytes at different passage number or ARF-depleted melanocytes were seeded in growth medium (M254 medium plus supplements) in XF96 V3 or XF24 V7 culture microplates (Seahorse Bioscience) at a density of 4.0 × 10 4 or 6.0 × 10 4 cells per well, respectively. OCR was investigated with the Seahorse XF96 or XF24 analyzer in growth medium following sequential additions of oligomycin (1 μM), FCCP (2.5 μM) and a combination of rotenone (2.5 μM) and antimycin A (2.5 μM). Pre-senescent melanocytes were electroporated twice with 2 μM NON-targeting smart pool siRNA (Dharmacon) or ARF-specific siRNA ( Supplementary Table 2 ) with a 24-h interval. Cells were seeded for Seahorse XF analysis 24 h after the last transfection. Tumour growth FM55-M2 melanoma cells were depleted of endogenous ARF and engineered to stably express EGFP, EGFP-ARF (wild type) or EGFP-ARF harbouring either the G65R, G65S or D68H mutations (see above). A total of 59 female NOG/NSG mice (Taconic) were subcutaneously injected in both flanks with 10 6 cells in a 100-μl 1:1 mixture of cell suspension and Geltrex (Invitrogen). In each group, mice were randomly assigned to one of two subgroups and, at the day after injection of cells, received intraperitoneal injections of 100 μl of PBS or a solution of 2-DG in PBS (100 mg ml −1 ) daily except for weekends. A total of 118 tumours were initially generated, distributed among 10 subgroups with at least 10 tumours in each. A total of 36 tumours were excluded from analysis either because of premature death of the mouse for unknown reason ( N =2), inability to fit tumour growth to an exponential model ( N =20) or signs of poor injections (multiple tumours at site of injection or abnormal tumour shape; N =14). Data analysis was based on growth profiles from 82 tumours. The time taken for each tumour to grow from a volume of 100 to 500 mm 3 was calculated based on the exponential equation descriptive of the growth of that tumour, leading to the calculation of a mean time for each group of PBS- or 2-DG-treated tumours. Ethics statement The handling of mice was conducted in accordance with the regulations set forward by the Danish Ministry of Justice and animal protection committees and in compliance with European Community Directive 86/609. Statistical analysis Data were analysed using WinSTAT version 2.0 software. Initial tests of normal distribution and variance homogeneity were performed using Kolmogorov–Smirnov and Bartlett’s tests, respectively, followed by one-way ANOVA. When necessary, data were either log10 or square root transformed to achieve normal distribution before ANOVA. Post hoc analysis was performed using LSD or Tukey tests. P values <0.05 were considered significant. How to cite this article : Christensen, C. et al . A short acidic motif in ARF guards against mitochondrial dysfunction and melanoma susceptibility. Nat. Commun. 5:5348 doi: 10.1038/ncomms6348 (2014).